Power laws reveal phase transitions in landscape controls of fire regimes Understanding the environmental controls on historical wildfires, and how they changed across spatial scales, is difficult because there are no surviving explicit records of either weather or vegetation (fuels). Here we show how power laws associated with fire-event time series arise in limited domains of parameters that represent critical transitions in the controls on landscape fire. Comparison to a self-organized criticality model shows that the latter mimics historical fire only in a limited domain of criticality, and is not an adequate mechanism to explain landscape fire dynamics, which are shaped by both endogenous and exogenous controls. Our results identify a continuous phase transition in landscape controls, marked by power laws, and provide an ecological analogue to critical behaviour in physical and chemical systems. This explicitly cross-scale analysis provides a paradigm for identifying critical thresholds in landscape dynamics that may be crossed in a rapidly changing climate. Nature displays power laws in frequency distributions of diverse phenomena [1] , [2] and critical exponents associated with phase transitions [3] , [4] . The latter are well known in thermodynamic and other physical systems, but in ecological systems they are more problematic to specify because of the complex dependencies associated with ecological dynamics [5] . Analyses of power-law behaviour in ecosystems frequently invoke self-organized criticality (SOC) [6] , [7] to explain how systems evolve to critical points. SOC has been suggested as an overarching mechanism for wildfire dynamics, as realized in a Forest Fire Model [8] (but see Loreto et al . [9] ), but it depends entirely on endogenous processes. In contrast, environmental controls on wildfires are thought to involve both fine-scale endogenous controls such as topography and spatial patterns of fuels and broader-scale (exogenous) drivers such as climate. We seek here to reconcile the potential for criticality to arise in wildfire regimes with the need to account for both endogenous and exogenous controls on fire spread. We use stochastic simulation and cross-scale analysis to quantify thresholds between these two types of controls in historical fire regimes. Fire-scarred trees provide a deep temporal record of fire activity in low-severity fire regimes [10] , [11] , [12] , wherein most trees survive, and record, most fires. We use this full spatio-temporal record to identify phase transitions in landscape fire between domains of endogenous versus exogenous control. The core of our analysis is a variogram-like metric, whose scaling behaviour follows power laws only when the fire regime is at a critical point. We provide an alternative interpretation of spatial patterns of fire to that of SOC by allowing for heterogenous landscape controls in the model, while explicitly modelling the phase transition between them. We use a spatially explicit fire-history database ( Fig. 1 ) with more than 7,000 fire-scarred trees. We replace the gamma statistic (semivariance) in a variogram with the Sørensen's distance [13] (SD), a multivariate measure of dissimilarity between pairs of time series of fires recorded in fire scars. The expectation of the SD variogram can be derived analytically from simple stochastic properties of fire spread and its memory in fire-scarred trees [14] . Power-law behaviour is evident in SD variograms from the most topographically complex watersheds, but clearly not in those with more simple topography ( Fig. 2 ). We deconstruct this power-law behaviour with a stochastic model based on exogenously constrained dynamic percolation (hereafter ECDP model), whose output replicates the SD variograms for each watershed. 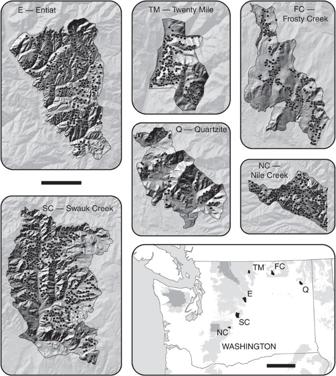Figure 1: Fire history study sites. Spatially explicit fire-scar records distributed across semi-arid mountain ecosystems of Washington, USA. Each point represents an individual recorder tree. The record extends back to the 1,500 s, but most trees in the database recorded a fire by 1,700, and there were few fires after 1,900, marking the onset of fire exclusion. We therefore used only data from 1,700 to 1,900 in this analysis. Fractal dimensions for each watershed (2—Hurst exponent from roughness-length regressions2) are Twenty Mile (1.20), Frosty Creek (1.25), Entiat (1.30), Nile Creek (1.33), Quartzite (1.35), Swauk Creek (1.40). Length of scale bar within index map is 100 km; length of scale bar for study area maps (E, TM, FC, SC, Q, NC) is 5 km. Figure 1: Fire history study sites. Spatially explicit fire-scar records distributed across semi-arid mountain ecosystems of Washington, USA. Each point represents an individual recorder tree. The record extends back to the 1,500 s, but most trees in the database recorded a fire by 1,700, and there were few fires after 1,900, marking the onset of fire exclusion. We therefore used only data from 1,700 to 1,900 in this analysis. Fractal dimensions for each watershed (2—Hurst exponent from roughness-length regressions [2] ) are Twenty Mile (1.20), Frosty Creek (1.25), Entiat (1.30), Nile Creek (1.33), Quartzite (1.35), Swauk Creek (1.40). Length of scale bar within index map is 100 km; length of scale bar for study area maps (E, TM, FC, SC, Q, NC) is 5 km. 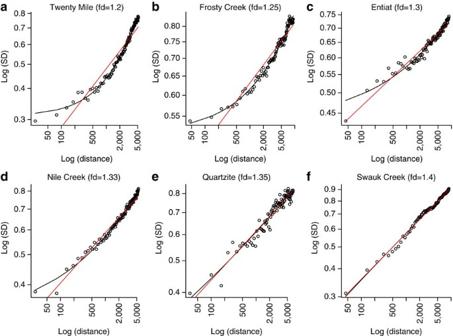Figure 2: Sørensen's distance variograms and power laws. Increasing power-law behaviour, as measured by linear fit of the SD variogram scatterplots in double logarithmic space, along a gradient of topographic complexity measured by fractal dimension (fd). Black lines are best-fit non-linear regression lines; red lines are the linear regressions (that is, power laws in log-log space). (a) Twenty Mile (b) Frosty Creek (c) Entiat (d) Nile Creek (e) Quartzite (f) Swauk Creek. Full size image Figure 2: Sørensen's distance variograms and power laws. Increasing power-law behaviour, as measured by linear fit of the SD variogram scatterplots in double logarithmic space, along a gradient of topographic complexity measured by fractal dimension (fd). Black lines are best-fit non-linear regression lines; red lines are the linear regressions (that is, power laws in log-log space). ( a ) Twenty Mile ( b ) Frosty Creek ( c ) Entiat ( d ) Nile Creek ( e ) Quartzite ( f ) Swauk Creek. Full size image The ECDP model simulates fire spread on a raster grid with three control parameters: p spread , the global probability that a cell burns after a neighbouring cell has burned, p scar , the probability that a recorder tree in the cell records the fire and μ size , the average maximum size a fire could attain (where individual fire sizes in the simulated fire history are drawn from a gamma probability distribution with mean= μ size ). p spread represents an endogenous control on fire spread, for example, the availability of fuel or a topographic barrier, and μ size represents an exogenous control, for example, the maximum duration of fire-conducive weather. The parameter p scar is the likelihood a tree that experiences fire records it with a scar, and fire spread is independent of this scarring probability. We asked whether a SOC model, which has been proposed to explain power laws in fire-size distributions [6] , can replicate the observed variability in the SD variograms. We built a simple 'forest fire' model [8] but added a CSR pattern (complete spatial randomness) of simulated recorder trees as in the ECDP model, so that a random draw determines whether a recorder tree that experiences fire records that fire with a scar. The SOC model is said to depend solely on emergent system properties, which self-organize to a critical state independently of exogenous driving forces, unlike the ECDP model, whose parameters are surrogates for both endogenous and exogenous drivers. Notably, the SOC model uses instantaneous spread (fires percolate deterministically), whereas the ECDP model tests via p spread at each cell, and percolation is a statistical property of the fire regime. Comparison of the ECDP model to the SOC model shows that the latter mimics historical fire only in a limited domain of criticality, and is not an adequate mechanism to explain landscape fire dynamics, which are shaped by both endogenous and exogenous controls. Our results identify a continuous phase transition in landscape controls between the purely endogenous and a mix of endogenous and exogenous controls, marked by power laws, and provide an ecological analogue to critical behaviour in physical and chemical systems. This explicitly cross-scale analysis provides a paradigm for identifying critical thresholds in landscape dynamics that may be crossed in a rapidly changing climate. Percolation threshold We found a percolation threshold for p spread , which is the value of p spread at which absent a size constraint, the first fire spans a suitably large raster grid. For our system we estimate this first fire spans at p spread =0.495. When we vary p spread between 0.35 and 1.0 and remove the size constraint, we find two domains in which simulated SD variograms follow power laws ( Fig. 3 ), one of which is centered on the percolation threshold, and represents a transition between fires that are mostly small and cannot propagate across a landscape and larger ones that can. This characterizes a phase transition in landscape dynamics over a narrow range of values for the parameter p spread , a region of criticality [15] , [16] in which we find that the SD variograms follow power laws. 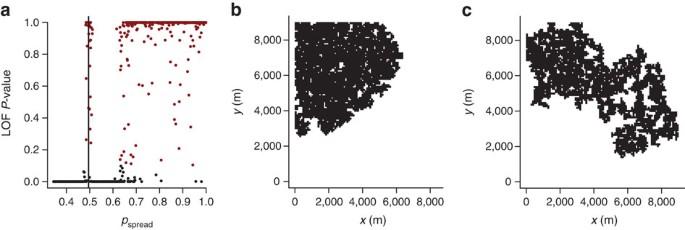Figure 3: Power laws at percolation threshold. Near the percolation threshold, power-law behaviour appears in the SD variogram in a narrow scaling region. This represents a phase transition between fires whose spread is endogenously controlled and those controlled by exogenous factors. (a) Power-law behaviour (linearity in log-log space) is apparent when a lack-of-fit (LOF) test for the linear model is not rejected (P-values between 0.10 and 1.0). Red dots indicateP≥0.1; black dots representP<0.1. A phase transition occurs atpspread≈0.495. Atpspread≥0.6, the LOF test is nonsignificant, but the result is trivial because the slope of the SD variogram is zero. This happens because for this part of the analysis we did not include exogenous controls on fire size. (b) Simulated fire shape withpspreadwell above the percolation threshold (0.57) shows a fire with a regular shape and a lower perimeter/area ratio. (c) Simulated fire shape withpspreadat or just below the threshold (0.49) shows a fire with an irregular shape and a higher perimeter/area ratio. Figure 3: Power laws at percolation threshold. Near the percolation threshold, power-law behaviour appears in the SD variogram in a narrow scaling region. This represents a phase transition between fires whose spread is endogenously controlled and those controlled by exogenous factors. ( a ) Power-law behaviour (linearity in log-log space) is apparent when a lack-of-fit (LOF) test for the linear model is not rejected ( P -values between 0.10 and 1.0). Red dots indicate P ≥0.1; black dots represent P <0.1. A phase transition occurs at p spread ≈0.495. At p spread ≥0.6, the LOF test is nonsignificant, but the result is trivial because the slope of the SD variogram is zero. This happens because for this part of the analysis we did not include exogenous controls on fire size. ( b ) Simulated fire shape with p spread well above the percolation threshold (0.57) shows a fire with a regular shape and a lower perimeter/area ratio. ( c ) Simulated fire shape with p spread at or just below the threshold (0.49) shows a fire with an irregular shape and a higher perimeter/area ratio. Full size image Interpretation of model parameters In the watersheds with the most complex topography, values of p spread that produce simulated SD variograms indistinguishable from the observed are very close to the percolation threshold, within the domain found to produce power-law SD variograms ( Fig. 4a ). The μ size parameter for these landscapes is ill-defined ( Fig. 4b ), as simulated fires fail to spread before the randomly drawn fire size is reached so that the simulated dynamics are independent of the value of μ size . The analogue to p spread could be a topographic barrier or a discontinuity of fuels, and we interpret that for landscapes with p spread near the percolation threshold, there is a balance between exogenous and endogenous controls on fire spread. 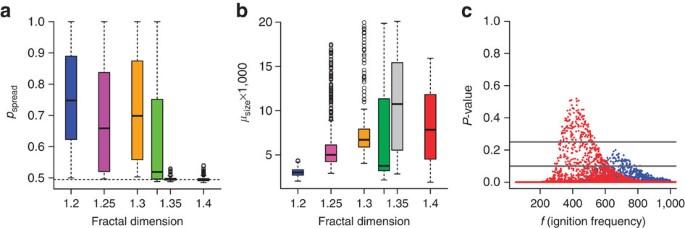Figure 4: Monte Carlo tests. Monte Carlo tests of parameters from the original stochastic model and the SOC model. (a) Distributions ofpspreadthat produced SD variograms not significantly different (α=0.25) from real watersheds, based on Monte Carlo simulations described in Methods. With increasing topographic complexity,pspreadapproaches the percolation threshold of 0.495. Watersheds left-to-right (also inb): Twenty Mile, Frosty Creek, Entiat, Nile Creek, Quartzite, Swauk Creek. (b) Distributions ofμsizethat produced SD variograms not significantly different (α=0.25) from real watersheds. In contrast topspread, the optimal value ofμsizeis more tightly constrained in watersheds of lower topographic complexity. Watersheds left-to-right: same as ina. (c) Distribution ofP-values for lack-of-fit tests of the ignition frequency parameter in the SOC model, showing a scaling region of nonsignificance (P>0.25) for Swauk Creek (red dots), with complex topography, but not for Twenty Mile (blue dots), and confirming that the SOC model replicates landscape fire dynamics only in the region of criticality. Theα-level (0.25) for these tests provides much more control of Type II error (that is, a rigorous matching of simulated to observed SD variograms) than classic experiments such as clinical trials or ecological field experiments, wherein control of Type I error is clearly paramount. Figure 4: Monte Carlo tests. Monte Carlo tests of parameters from the original stochastic model and the SOC model. ( a ) Distributions of p spread that produced SD variograms not significantly different ( α =0.25) from real watersheds, based on Monte Carlo simulations described in Methods. With increasing topographic complexity, p spread approaches the percolation threshold of 0.495. Watersheds left-to-right (also in b ): Twenty Mile, Frosty Creek, Entiat, Nile Creek, Quartzite, Swauk Creek. ( b ) Distributions of μ size that produced SD variograms not significantly different ( α =0.25) from real watersheds. In contrast to p spread , the optimal value of μ size is more tightly constrained in watersheds of lower topographic complexity. Watersheds left-to-right: same as in a . ( c ) Distribution of P -values for lack-of-fit tests of the ignition frequency parameter in the SOC model, showing a scaling region of nonsignificance ( P >0.25) for Swauk Creek (red dots), with complex topography, but not for Twenty Mile (blue dots), and confirming that the SOC model replicates landscape fire dynamics only in the region of criticality. The α -level (0.25) for these tests provides much more control of Type II error (that is, a rigorous matching of simulated to observed SD variograms) than classic experiments such as clinical trials or ecological field experiments, wherein control of Type I error is clearly paramount. Full size image In contrast, as topographic complexity lessens, the distribution of p spread values able to replicate observed SD variograms converges well above the percolation threshold ( Fig. 4a ). The μ size parameter is well defined for these landscapes because the simulated fires require the random fire size-based stopping rule in order to not span the raster grid ( Fig. 4b ). For p spread well above the percolation threshold, changes in the p spread parameter have diminished effects, and the shape of the SD variogram is more sensitive to changes in the μ size parameter, such that the balance is shifted towards exogenous controls. Comparison to SOC model By tuning the ratio of frequency of ignitions to fuel accumulation, as in the original SOC model, we sought to replicate the observed SD variograms in the two watersheds with the most contrasting topographic complexity: Swauk Creek and Twenty Mile. We find that whereas the SOC model can replicate the spatial structure (and power-law behaviour) recorded in the SD variogram for Swauk Creek, with complex topography, in the watershed with the simplest topography (Twenty Mile) it does not ( Fig. 4c ). Two inferences arise from the failure of SOC to replicate observed behaviour except at criticality. First, SOC cannot predict the scaling region surrounding the phase transition we discovered and explained with the ECDP model; second, SOC is therefore an incomplete representation of processes that drive real fire regimes across landscapes, except perhaps at precisely the parameter values where dynamics are in a domain of criticality. Furthermore, it is even less likely that SOC is globally justified as a mechanism for fire-size distributions across an entire region [17] , where fires do not experience the same environmental controls, nor do they influence each other's behaviour and spread. The underlying assumption of SOC is that the endogenous processes controlling fire on real landscapes operate in a region of criticality. Not surprisingly then, the dynamics of SOC overlap with the ECDP model near the percolation threshold (also a region of criticality). We show that this region applies to watersheds with complex topography, but not to watersheds with simpler topography. Unlike SOC, ECDP finds a transition between sites where the endogenous controls (for example, topographic constraints) balance exogenous forcings (for example, fire weather) [18] and sites where exogenous forcings have a greater impact. Although SOC may indeed be a mechanism producing power-law behaviour, on real landscapes it operates only within the phase transition we have identified. A further inference is that the SD variogram not only provides more information about historical fires than (reconstructed) fire-size distributions, but also is a more sensitive and robust indicator of criticality [15] . Universal explanations are rare in ecological phenomena. They generally fail to be consistent with observations except in limited domains. A simple stochastic model (ECDP), in conjunction with scaling laws as manifest in the SD variogram, has identified a scaling region with strong parallels to phase transitions in the physical sciences, but the difference is that this domain of criticality is embedded in complex causal dependencies characteristic of ecological systems [5] . For example, our phase transition is fairly abrupt in units of the stochastic parameter p spread, but spans a broader scaling region in more standard units of topographic complexity, for example, fractal dimension. The strength of power-law behaviour in the observed SD variograms ( Fig. 2 ) is strongly correlated with the estimated fractal dimensions of the watersheds [19] . We would expect this scaling region to shift with stronger exogenous forcing, such as the increased flammability and more intense fire behaviour in a hotter and drier climate. Under such conditions topography would have to be even more complex for fire dynamics to remain at the phase transition. Quantifying the transition between endogenous and exogenous controls on landscape fire should improve predictions of the response of fire regimes to a rapidly changing climate [20] . The power-law domain found in SD variograms is a surrogate for the interactions of multiple processes at criticality (for example, fire weather, topographic constraints and their effect on fuel configurations, tree scarring by fire), all of which can be measured only with considerable error and whose future patterns are uncertain. In this study, the power-law domain observed at the balance of exogenous and endogenous controls represents the climate during the time domain of the fire history (1,700–1,900). Topography (hence endogenous control) remains relatively constant, but future climate will not, disturbing the balance of exogenous and exogenous controls, such that topographies for which power-law SD variograms apply historically may not produce them in the future. If exogenous controls on fire spread strengthen in the future (for example, more extreme fire weather), then one might expect a shift in the shape of the SD variogram for complex landscapes to that observed for the simpler landscapes, effectively increasing the p spread value and moving the system away from the phase transition. By overlaying barriers to fire spread at judiciously chosen coordinates [21] , however, to mimic increasing topographic complexity (artificially increasing the fractal dimension of the landscape), we may discover simple but robust treatments to maintain fire-adapted landscapes that are resilient to climate change. Fire-history data Fire-history reconstructions in low-severity fire regimes rely on the presence of fire-scarred trees (recorder trees) in a landscape, where the presence of a scar is cross-dated to provide an estimate of the year and sometimes season in which a fire occurred. Our data set records not only the presence of scars, but also the locations of the recorder trees. This data set provides a marked point pattern of recorder trees, with the marks being the observation of a scar a given year. A fire-history matrix summarizes the scar pattern for a set of recorder trees in a given landscape ( Supplementary Table S1 ). For each combination of tree and fire year an entry in the matrix is 1, if the tree records that fire, and 0 otherwise. The Sørensen distance variogram We calculated the SD for every pair of recorder trees on a given landscape. The SD is a semimetric commonly used in community ecology to measure species co-occurrence. It is calculated from a frequency table that compares the fire history of two recorder trees ( Supplementary Table S2 ; equation (1)) SD can take continuous values on the range (0,1), with zero indicating completely similar fire histories between a pair of trees and one indicating completely dissimilar fire histories between a pair of trees. The choice of SD was motivated by a remarkably elegant relationship between its expectation (E[SD]) and the probabilistic nature of recorder-tree scarring. Kennedy and McKenzie [14] used the probability structure implicit in ECDP to derive an expectation for the value of SD between a given pair of recorder trees (A and B) ( Supplementary Table S3 ). When combined algebraically, the complicated equations in Supplementary Table S3 reduce to a simple expression for the expected value of SD (3). where P(B fire |A fire ) is the probability a second tree (B) experiences fire given the first tree (A) has experienced fire. This probability depends on the spatial structure of the fire and the fire size, which change with the model parameters p spread and μ size . Therefore, the shape of the SD variogram depends on the fire size and the spatial structure of fire spread, connecting the SD variogram directly to the spatio-temporal pattern in a fire history. SD variograms are produced by binning the between-tree pairwise geographic distances, calculating the mean SD for all pairs of trees for a given distance bin, and plotting the mean SD against geographic distance. We truncate the SD variogram at half the maximum geographic distance between recorder trees, following the paradigm for variogram analysis in spatial ecology. Beyond this distance, variograms typically have sample sizes in bins that are too small, and outliers will confound inferences [22] . ECDP model ECDP simulates two processes: fire spread and recorder tree scarring ( Supplementary Fig. S1 ). ECDP is initialized with a blank raster grid with 100×100 pixels. A point pattern of CSR recorder trees is overlain on the raster grid and retained throughout the simulated fire history. These are the trees available for scarring, and fire spread is independent of the presence of recorder trees. The number of fires simulated for an individual is a random number determined by sequential draws from an exponential distribution. For each fire in the history, a random fire size expressed as the number of pixels burned is drawn from a gamma distribution whose mean is a mean fire size ( μ size ). For each fire, an ignition point on the raster grid is randomly chosen, with a five-cell buffer excluded along the edge. Fire spreads iteratively from the ignition point according to a simple probability test ( p spread ; Supplementary Fig. S1 ). For each fire in the history, this process is iterated until one of three stopping points is reached. (1) If all tests of spread fail in a given iteration, the fire can no longer spread and the next fire is initialized (the fire burns out on its own). (2) If the number of pixels burned in the current fire is more than the random fire size, then fire spread is halted and the next fire is initialized. (3) If the fire spreads to each of the four borders of the raster grid before the fire reaches its random size, fire spread is halted and the next fire is initialized. Each fire is spread independently of the previous fires, so there is no memory in the landscape process. For details of the ECDP model, see ref. 2 . SOC model with fire scars We programmed an SOC forest fire model ( Supplementary Fig. S2 ) after Malamud et al . [6] and overlaid a CSR pattern of recorder trees on the SOC grid. The SOC model is initialized with a blank raster grid. At each iteration, fuel is dropped randomly on the grid, with each pixel having an equal chance to receive fuel. The tunable parameter of the SOC model is the frequency of sparks that are dropped onto the SOC grid ( f ). In our version, fuel accumulation and sparking are independent of the presence of recorder trees, which occupy a given pixel throughout the simulated fire history. If a pixel included in the SOC fire is occupied by a recorder tree, then that tree is tested for scarring as in the ECDP model. Our modified SOC model then has two parameters: frequency of sparks ( f ) and probability of scarring ( p scar ). Details of the SOC fire model are in many recent publications [7] , [8] . Monte Carlo tests for SD variograms This study was motivated by the variability in the shape of the SD variogram across landscapes with varying topography. Rather than inferring directly from these patterns, we use Monte Carlo inference to test whether a stochastic model (ECDP) can replicate the observed variability. We use spatially explicit simulations to remove biases associated with mean-field approximations of spatial processes, which can confound the identification of critical thresholds [23] . The model parameters are surrogates for underlying ecological processes; for example, p spread is interpreted as endogenous controls on fire spread, and μ size is interpreted as exogenous controls on fire spread. If a model is found that can replicate the variability in observed patterns, we use the interpretation of the model parameters that corresponds to the observed pattern for each landscape to infer its dominant controls. It is therefore the correspondence of the model to the observed patterns (that is, each is driven by a spatial process), through the Monte Carlo inference procedure, that enables the major conclusions to be drawn. We used the ECDP model to produce simulated SD variograms and evaluated how well it can replicate the observed SD variograms using a Monte Carlo goodness-of-fit procedure [24] , which tests the hypothesis: is the observed pattern a typical model realization? For each site, this procedure returns the set of combinations of p spread , p scar and μ size that cannot be rejected relative to the observed pattern. We used an analogous procedure to evaluate the SOC model, finding the combinations of frequency of sparks ( f ) and probability of scarring ( p scar ) that cannot be rejected. A significance level of 0.25 was set for both, given that a primary concern was to control for Type II error (overly liberal acceptance of the replication of observed SD variograms by the models). Identifying the phase transition To quantify the region of criticality, we evaluated domains of p spread over which the ECDP model produces power-law SD variograms. First, we sampled 1,000 values of p spread uniformly on (0,1). We set the ECDP model to remove the size-based stopping rule, thereby isolating the effect of p spread on the shape of the SD variogram. For each value of p spread , we conducted 20 replicate simulations, yielding 20 simulated SD variograms for each value of p spread . We then used the replicate simulations in an F -test for lack-of-fit to determine whether the power law can be rejected for the simulated SD variograms with the associated value of p spread . The significance level was 0.10—a more balanced consideration of Type I versus Type II errors because regions in which power laws occurred and where they did not were both of interest. In reality, only one point near the percolation threshold fell between P =0.10 and 0.25 ( Fig. 3 ). How to cite this article: McKenzie, D. & Kennedy, M.C. Power laws reveal phase transitions in landscape controls of fire regimes. Nat. Commun. 3:726 doi: 10.1038/ncomms1731 (2012).